Mutations inDYNC2LI1disrupt cilia function and cause short rib polydactyly syndrome The short rib polydactyly syndromes (SRPSs) are a heterogeneous group of autosomal recessive, perinatal lethal skeletal disorders characterized primarily by short, horizontal ribs, short limbs and polydactyly. Mutations in several genes affecting intraflagellar transport (IFT) cause SRPS but they do not account for all cases. Here we identify an additional SRPS gene and further unravel the functional basis for IFT. We perform whole-exome sequencing and identify mutations in a new disease-producing gene, cytoplasmic dynein-2 light intermediate chain 1, DYNC2LI1 , segregating with disease in three families. Using primary fibroblasts, we show that DYNC2LI1 is essential for dynein-2 complex stability and that mutations in DYNC2LI1 result in variable length, including hyperelongated, cilia, Hedgehog pathway impairment and ciliary IFT accumulations. The findings in this study expand our understanding of SRPS locus heterogeneity and demonstrate the importance of DYNC2LI1 in dynein-2 complex stability, cilium function, Hedgehog regulation and skeletogenesis. The primary cilium is a microtubule-based projection on the surface of nearly every cell that acts as a concentrated signalling centre for several pathways [1] . Defects in the formation or function of primary cilia cause a wide variety of disorders known as ciliopathies. As a testament to the importance of this organelle, ciliopathies collectively affect all major organ systems [2] , including the skeleton. Cilium assembly and function require intraflagellar transport (IFT), a system for bidirectional traffic into and out of this organelle. IFT depends on the microtubule motor protein activities of two multi-protein complexes [3] : IFT-B, the kinesin-2-driven anterograde complex, mediates base-to-tip transport, and IFT-A, the dynein-2-driven retrograde complex, mediates tip-to-base transport. The SRPSs are autosomal recessive, perinatal lethal disorders. Radiographic abnormalities include very short, horizontal ribs, short limbs and variable degrees of polydactyly. Other organ system abnormalities, particularly those affecting the heart and kidney, are frequently seen. SRPSs are part of a spectrum of heterogeneous skeletal ciliopathies that include asphyxiating thoracic dystrophy, Ellis van Creveld and Sensenbrenner syndromes. Mutations in the gene encoding the IFT-A cytoplasmic dynein-2 motor heavy chain, DYNC2H1 (MIM 603297), are the most common cause of both SRPS and asphyxiating thoracic dystrophy [4] , [5] . Recently, mutations in several additional genes have been shown to cause SRPS: IFT80 (refs 6 , 7 ; MIM 611263), WDR35 (refs 8 , 9 ; MIM 614091), WDR19 (ref. 10 ; MIM 614376), NEK1 (refs 11 , 12 ; MIM 263520), WDR34 (refs 13 , 14 ; MIM 615633), IFT140 (refs 15 , 16 ; MIM 266920), IFT172 (ref. 17 ; MIM 615630), WDR60 (ref. 18 ; MIM 615462) and TTC21B [19] (MIM 612014). Among the proteins encoded by the SRPS genes, WDR60 and WDR34 are intermediate chains of the DYNC2H1 cytoplasmic dynein-2 complex, highlighting its importance in skeletal development [20] . Here we show that mutations in another member of the complex, DYNC2LI1 , also cause SRPS, in part through loss of complex stability. The IFT-A dynein-2 complex is composed of at least five components: the dynein heavy chain DYNC2H1 (DHC1b) [21] , [22] , [23] , the two intermediate chains WDR34 (DIC5/FAP133; ref. 24 ) and WDR60 (FAP153; ref. 25 ), the light intermediate chain DYNC2LI1 (D1bLIC/D2LIC/LIC3/XBX1; refs 26 , 27 , 28 , 29 ) and the LC8 light chain [30] . DYNC2LI1 was described as a novel dynein light intermediate chain based on its amino acid sequence, its ability to interact with DYNC2H1 and its localization to cilia [26] , [31] . As an accessory chain binding to the base of the dynein-2 complex, DYNC2LI1 is likely involved in tethering the dynein-2 motor to substrates such as vesicles and providing docking sites for cargo [26] , [31] . It is essential for ciliogenesis and contains an X-box promoter that is recognized by the ciliary transcription factor RFX3/DAF-19 (refs 28 , 32 ). Recent studies have shown that DYNC2LI1 is essential for dynein-2 complex stability and its depletion in Trypanosoma brucei and Chlamydomonas reinhardtii results in loss and mislocalization of DYNC2H1 (refs 24 , 29 , 33 , 34 ). Furthermore, DYNC2LI1 mouse mutants result in lethality early in embryogenesis with developmental abnormalities characteristics of severe Hedgehog signalling defects [35] . In this study, we identify mutations in DYNC2LI1 causing SRPS in three independent cases. We show that DYNC2LI1 is essential for dynein-2 complex stability, is expressed in the cartilage growth plate and plays critical roles in the regulation of primary cilium length, retrograde IFT and Hedgehog signalling. Analysis of SRPS-derived fibroblasts supports a role for DYNC2LI1 in cilia function and signalling and the findings highlight the importance of this gene and the dynein-2 complex in skeletogenesis. DYNC2LI1 mutations identified in SRPS cases To identify additional genes that are essential for skeletal development, we used whole-exome sequencing under an approved human subjects protocol and identified mutations in the dynein-2 light intermediate chain gene, DYNC2LI1 , producing SRPS. Three probands from unrelated Caucasian families were identified by prenatal ultrasound, and elective terminations were performed at 14, 19 and 22 weeks, respectively. In the prenatal period, ultrasound findings included shortened long bones, diminished chest circumferences for gestational age and polydactyly. No other obvious organ system abnormalities were detected by ultrasound. Radiographic analyses showed polydactyly of the upper and lower extremities, a long narrow thorax with very short horizontal ribs, lack of ossification of some skeletal elements and irregular metaphyseal borders with lateral spikes ( Fig. 1 ). These findings are characteristics of SRPS and radiographically similar to SRPS cases described with DYNC2H1 and WDR34 mutations [4] , [13] , [36] . 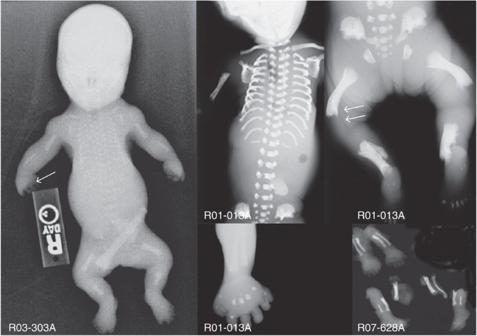Figure 1: Mutations inDYNC2LI1cause SRPS. Radiographs of the affected probands, R03-303A, R01-013A and R07-628A (International Skeletal Dysplasia Registry reference numbers) showing short long bones, horizontal ribs and long narrow chest, poor mineralization of some skeletal elements (single arrow), metaphyseal irregularity (double arrows) and polydactyly in all the limbs of the affected individuals. Figure 1: Mutations in DYNC2LI1 cause SRPS. Radiographs of the affected probands, R03-303A, R01-013A and R07-628A (International Skeletal Dysplasia Registry reference numbers) showing short long bones, horizontal ribs and long narrow chest, poor mineralization of some skeletal elements (single arrow), metaphyseal irregularity (double arrows) and polydactyly in all the limbs of the affected individuals. Full size image In all three cases there was compound heterozygosity for mutations in DYNC2LI1 ( Supplementary Fig. 1 ). Two affected individuals, R01-013A and R03-303A, were heterozygous for changes in intron 12 (c.993+1G>A, c.993+3A>G) that are predicted to affect splicing ( Table 1 ). RT–PCR (PCR with reverse transcription) analysis on RNA derived from fibroblasts from both fetuses demonstrated that both mutations resulted in in-frame skipping of exon 12 ( Fig. 2a ). R01-013A and R07-628A were both heterozygous for a point mutation causing the predicted amino acid p.Leu117Val substitution. This missense mutation occurs within a region conserved among the three mammalian dynein light intermediate chains and resides within an NTPase-related domain ( Supplementary Fig. 2 ). This mutation may interfere with cargo-binding as it occurs within a homologous region that is required for cargo-binding in DYNC1LI1 (ref. 37 ). However, of the three mammalian dynein light intermediate chains, only DYNC2LI1 interacts with the dynein-2 complex; the more closely related DYNC1LI1 and DYNC1LI2 are targeted to the non-ciliary cytoplasmic dynein-1, DYNC1H1 (refs 26 , 38 ). Finally, the other heterozygous changes in R07-628A and R03-303A were nonsense mutations in exon 6 (p.Trp124Ter) and 13 (p.Glu334Ter), respectively. Western blot analyses of fibroblast-derived lysates showed that DYNC2LI1 is markedly reduced in R01-013A (c.993+1G>A; p.Leu117Val) and R07-628A (p.Trp124Ter; p.Leu117Val), indicating that these mutations likely lead to loss of DYNC2LI1 stability ( Fig. 2b,c ). Table 1 Pathogenic DYNC2LI1 mutations in SRPS cohort. 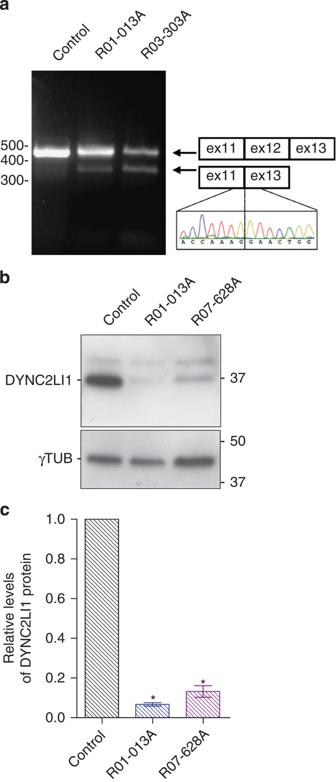Figure 2: Effect ofDYNC2LI1mutations on splicing and protein stability. (a) RT–PCR of cDNA derived from control and SRPS fibroblasts shows thatDYNC2LI1splice-donor mutations cause in-frame skipping of exon 12. (b) Immunoblotting reveals significant reduction in the amounts of DYNC2LI1 from lysates of affected cells compared with control. Size markers (right, kDa), γ-tubulin, loading control. (c) Quantification of average DYNC2LI1 amounts from (b) for each genotype. Values were normalized to control and error bars represent±s.e.m (three independent experiments). Statistical analyses were performed using the Mann–Whitney test, *P<0.05. Full size table Figure 2: Effect of DYNC2LI1 mutations on splicing and protein stability. ( a ) RT–PCR of cDNA derived from control and SRPS fibroblasts shows that DYNC2LI1 splice-donor mutations cause in-frame skipping of exon 12. ( b ) Immunoblotting reveals significant reduction in the amounts of DYNC2LI1 from lysates of affected cells compared with control. Size markers (right, kDa), γ-tubulin, loading control. ( c ) Quantification of average DYNC2LI1 amounts from ( b ) for each genotype. Values were normalized to control and error bars represent±s.e.m (three independent experiments). Statistical analyses were performed using the Mann–Whitney test, * P <0.05. Full size image DYNC2LI1 -mutant fibroblasts are depleted of DYNC2H1 DYNC2H1 and DYNC2LI1 are distinct components of the ciliary dynein-2 complex, and studies in C. reinhardtii and T. brucei show that loss of one results in loss or reduction of the other [24] , [29] , [33] , [34] . To determine whether DYNC2H1 amounts were affected by the decrease in DYNC2LI1, we probed whole-cell lysates from SRPS cases and controls for DYNC2H1 and discovered near-total loss of protein ( Fig. 3a ). The amounts of the dynein-2 intermediate chain WDR34 and the heavy chain of the dynein-1 complex (DYNC1H1) were unchanged, indicating that the effects of the DYNC2LI1 mutations were specific to DYNC2H1. Immunofluorescence staining showed that WDR34 and the minimal remaining DYNC2H1 in SRPS cells localized to the basal bodies, similar to controls ( Fig. 3b ). These results suggest that even though DYNC2LI1 is important for the stabilization of DYNC2H1, it is not essential for the recruitment of the dynein-2 complex to the pericentriolar region of basal bodies. 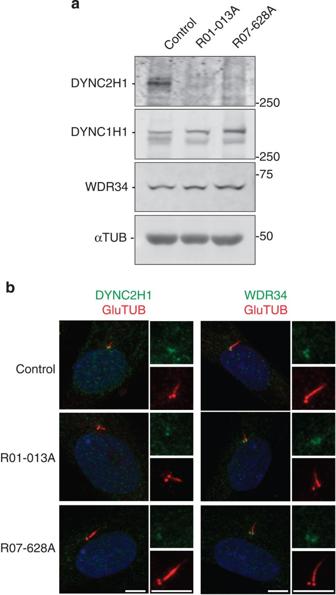Figure 3: Mutations inDYNC2LI1decrease the stability of DYNC2H1. (a) Immunoblotting for components of the dynein-2 complex (heavy chain, DYNC2H1; intermediate chain, WDR34) and the heavy chain of the dynein-1 complex (DYNC1H1) reveals a specific reduction of DYNC2H1. (b) Immunofluorescence micrographs of control and SRPS cells stained for GluTUB (red) and WDR34 (green) or DYNC2H1 (green). Cilia (2 × ) are shown on the right. Scale bar, 5 μm. Figure 3: Mutations in DYNC2LI1 decrease the stability of DYNC2H1. ( a ) Immunoblotting for components of the dynein-2 complex (heavy chain, DYNC2H1; intermediate chain, WDR34) and the heavy chain of the dynein-1 complex (DYNC1H1) reveals a specific reduction of DYNC2H1. ( b ) Immunofluorescence micrographs of control and SRPS cells stained for GluTUB (red) and WDR34 (green) or DYNC2H1 (green). Cilia (2 × ) are shown on the right. Scale bar, 5 μm. Full size image DYNC2LI1 is expressed in the developing human growth plate While the dynein-2 complex is required for IFT in all ciliated cells of the body, the marked skeletal consequences of dynein-2 complex mutations suggest that the developing skeleton is very sensitive to reductions in its activity. Concordant with this hypothesis, transcriptional analysis by quantitative RT–PCR (qRT–PCR) showed that DYNC2LI1 was more highly expressed in bone compared with other embryonic tissues (bone, brain, cartilage, heart, liver, lung, placenta and thymus; Supplementary Fig. 3 ). Furthermore, immunohistochemistry of human cartilage growth plate revealed DYNC2LI1 expression in the perichondrium, periosteum and primary spongiosa of bone ( Fig. 4 ). Similarly, immunohistochemistry of DYNC2H1 and WDR34 showed an overlapping expression pattern ( Fig. 4 ). Together, these expression studies support a role for DYNC2LI1 and the dynein-2 complex in human skeletal development. 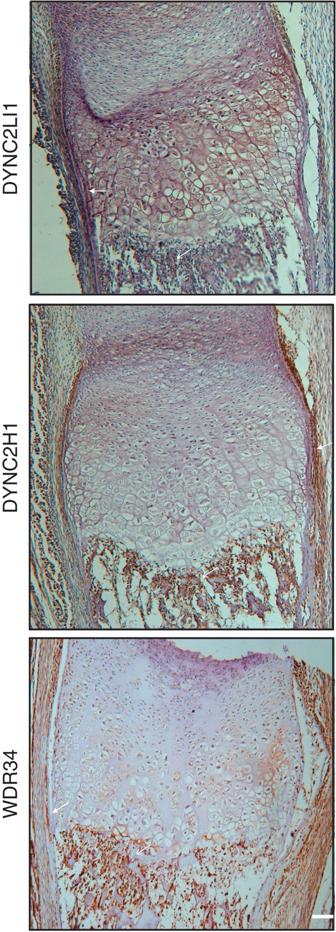Figure 4: Components of the dynein-2 complex are co-expressed in a human cartilage growth plate. (a) Sections from a 14-week human humerus were stained for DYNC2LI1, DYNC2H1 and WDR34. All three proteins were expressed in the perichondrium/periosteum and primary spongiosa (closed arrows, perichondrium/periosteum; open arrows, primary spongiosa). Scale bar, 50 μm. Figure 4: Components of the dynein-2 complex are co-expressed in a human cartilage growth plate. ( a ) Sections from a 14-week human humerus were stained for DYNC2LI1, DYNC2H1 and WDR34. All three proteins were expressed in the perichondrium/periosteum and primary spongiosa (closed arrows, perichondrium/periosteum; open arrows, primary spongiosa). Scale bar, 50 μm. Full size image SRPS fibroblasts exhibit loss of ciliary length control To investigate whether mutations in DYNC2LI1 affect ciliogenesis and/or IFT, we quantified the fraction of ciliated cells, measured cilia length and probed SRPS and control fibroblasts for a number of ciliary components. The percentage of ciliated cells was only slightly reduced between SRPS and control cells ( Fig. 5b ). However, we found that primary cilia length was highly variable in SRPS fibroblasts, with a substantial increase in the number of hyperelongated cilia up to 20 μm in length ( Fig. 5a,c,d ). To determine whether the ciliary length variation observed in SRPS cells resulted from decreased amounts of DYNC2LI1, we performed RNAi against DYNC2LI1 in hTERT–RPE1 (retinal epithelial) cells. DYNC2LI1 knockdown led to significantly increased variation in cilia length, thus reproducing the phenotype observed in SRPS fibroblasts ( Supplementary Fig. 4a,b ). To test for phenotypic rescue, we expressed wild-type DYNC2LI1 in SRPS cells. As shown in Fig. 5c,d , transfection of DYNC2LI1 into SRPS fibroblasts reduced ciliary length variation and restored length to control values. We therefore conclude that DYNC2LI1 and the dynein-2 complex play an important role in the regulation of primary cilia length. 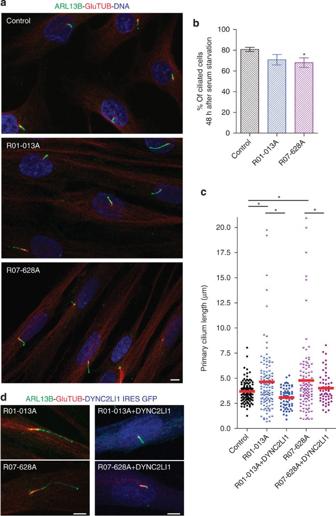Figure 5: Primary cilia are variable in length and longer inDYNC2LI1-mutant cells. (a) Immunofluorescence micrographs of serum-starved control and SRPS fibroblasts stained for ARL13B (green), GluTUB (red) and Hoescht (blue) show variable length and hyperelongated cilia in SRPS cells. (b) Percentage of ciliated cells in (a) (n=150 × 3 independent experiments). (c) Primary cilia length is highly variable in cells withDYNC2LI1mutations (n>20 × 3 independent experiments). (d) Expression of untagged wild-type DYNC2LI1 through an IRES-GFP vector (artificially coloured blue) rescues cilia length variability in SRPS cells. Error bars represent±s.e.m. Statistical analyses performed using Mann–Whitney test, *P<0.05. Scale bar, 5 μm. Figure 5: Primary cilia are variable in length and longer in DYNC2LI1 -mutant cells. ( a ) Immunofluorescence micrographs of serum-starved control and SRPS fibroblasts stained for ARL13B (green), GluTUB (red) and Hoescht (blue) show variable length and hyperelongated cilia in SRPS cells. ( b ) Percentage of ciliated cells in ( a ) ( n =150 × 3 independent experiments). ( c ) Primary cilia length is highly variable in cells with DYNC2LI1 mutations ( n >20 × 3 independent experiments). ( d ) Expression of untagged wild-type DYNC2LI1 through an IRES-GFP vector (artificially coloured blue) rescues cilia length variability in SRPS cells. Error bars represent±s.e.m. Statistical analyses performed using Mann–Whitney test, * P <0.05. Scale bar, 5 μm. Full size image IFT components accumulate in DYCN2LI1 -mutant cilia The IFT-B components, IFT88 and TRAF3IP1, and the IFT-B kinesin motor, KIF3A, localized strongly to the base of the cilia and weakly along the axoneme in control cells, as observed by others [39] ( Fig. 6a ). Consistent with defective retrograde transport in SRPS fibroblasts, IFT88, TRAF3IP1 and KIF3A all accumulated near the cilia tip. More specifically, three- to four-fold more IFT88 was retained in the axonemes of DYNC2LI1 -mutant cilia than in controls ( Fig. 6c ). RNAi knockdown of DYNC2LI1 in RPE1 cells replicated this finding by increasing the ratio of IFT88 retained in the primary cilium body relative to the proximal end by threefold ( Supplementary Fig. 4c,d ). In addition, we were able to reduce this ratio in SRPS fibroblasts by expressing wild-type DYNC2LI1 ( Fig. 6b,c ). Our results demonstrate that loss of DYNC2LI1 markedly impairs retrograde IFT and leads to the accumulation of IFT proteins within the primary cilium. 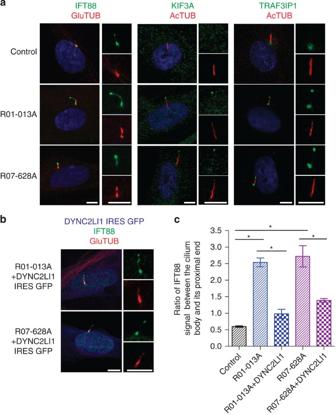Figure 6:DYNC2LI1mutations delay retrograde IFT and lead to the ciliary accumulation of IFT components. (a) Immunofluorescence micrographs of control and SRPS cells stained as labelled. Cilia (2 × ) are shown on the right. (b) Expression of untagged wild-type DYNC2LI1 through an IRES-GFP vector (artificially coloured blue) rescues ciliary accumulation of IFT components. (c) Quantification of IFT88 signal: graph shows the mean ratio of IFT88 signal between the cilium body and its proximal end±s.e.m (n=20 × 3 independent experiments). Statistical analyses were performed using Mann–Whitney test, *P<0.05. Scale bar, 5 μm. Figure 6: DYNC2LI1 mutations delay retrograde IFT and lead to the ciliary accumulation of IFT components. ( a ) Immunofluorescence micrographs of control and SRPS cells stained as labelled. Cilia (2 × ) are shown on the right. ( b ) Expression of untagged wild-type DYNC2LI1 through an IRES-GFP vector (artificially coloured blue) rescues ciliary accumulation of IFT components. ( c ) Quantification of IFT88 signal: graph shows the mean ratio of IFT88 signal between the cilium body and its proximal end±s.e.m ( n =20 × 3 independent experiments). Statistical analyses were performed using Mann–Whitney test, * P <0.05. Scale bar, 5 μm. Full size image SMO inappropriately enters the cilia of SRPS fibroblasts Hedgehog signalling requires intact cilia and IFT; not surprisingly, many IFT mutants display defects in this pathway [40] . To determine whether DYNC2LI1 mutations affect Hedgehog signalling, we examined the localization of smoothened, frizzled class receptor (SMO) and GLI3 in SMO agonist (SAG)-stimulated and -unstimulated fibroblasts from SRPS cases and controls. While the localization of GLI3 did not differ between SRPS and control cells ( Fig. 7a ), we detected SMO along the length of cilia of unstimulated DYNC2LI1 -mutant cells ( Fig. 7b,c ). In contrast, SMO was only observed in the cilia of control cells upon stimulation. Similar to findings in DYNC2H1 mouse mutants [41] , these observations suggest that DYNC2LI1 and the activity of the dynein-2 complex play an important role in preventing SMO from entering cilia in the absence of Hedgehog stimulation. 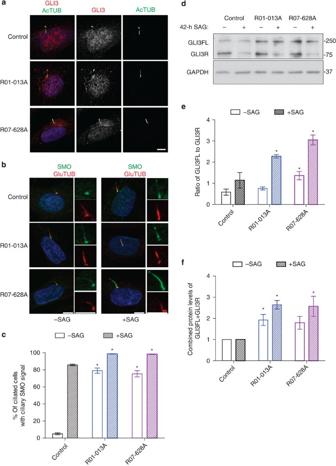Figure 7: Disruption of the dynein-2 complex leads to aberrant Hedgehog signalling. (a) Immunofluorescence micrographs of control and SRPS cells treated with SAG and stained for GLI3 (red), AcTUB (green) and 4,6-diamidino-2-phenylindole (blue). (b) DYNC2LI1/dynein-2 complex activity is required for the exclusion of SMO from the primary cilium in the absence of Hedgehog stimulation. Immunofluorescence micrographs of SAG-stimulated control and SRPS cells stained for SMO (green) and GluTUB (red). (c) Graph shows the mean percentage of ciliated cells with ciliary SMO±s.e.m. (>100 cells counted × three independent experiments). (d) Immunoblotting for GLI3 (full-length ‘GLI3FL’; repressor ‘GLI3R’) in cell extracts shows increased GLI3FL to GLI3R in SRPS cells. (e) Graph shows the ratio of GLI3FL to GLI3R. (f) Graph shows quantification of total GLI3 amounts (GLI3FL+GLI3R), which is increased inDYNC2LI1-mutant fibroblasts. Statistical analyses performed using Mann–Whitney test, *P<0.05. Scale bars, 5 μm. Figure 7: Disruption of the dynein-2 complex leads to aberrant Hedgehog signalling. ( a ) Immunofluorescence micrographs of control and SRPS cells treated with SAG and stained for GLI3 (red), AcTUB (green) and 4,6-diamidino-2-phenylindole (blue). ( b ) DYNC2LI1/dynein-2 complex activity is required for the exclusion of SMO from the primary cilium in the absence of Hedgehog stimulation. Immunofluorescence micrographs of SAG-stimulated control and SRPS cells stained for SMO (green) and GluTUB (red). ( c ) Graph shows the mean percentage of ciliated cells with ciliary SMO±s.e.m. (>100 cells counted × three independent experiments). ( d ) Immunoblotting for GLI3 (full-length ‘GLI3FL’; repressor ‘GLI3R’) in cell extracts shows increased GLI3FL to GLI3R in SRPS cells. ( e ) Graph shows the ratio of GLI3FL to GLI3R. ( f ) Graph shows quantification of total GLI3 amounts (GLI3FL+GLI3R), which is increased in DYNC2LI1 -mutant fibroblasts. Statistical analyses performed using Mann–Whitney test, * P <0.05. Scale bars, 5 μm. Full size image DYNC2LI1 mutants exhibit reduced GLI3 processing To further investigate Hedgehog pathway activation, we measured GLI3 processing in affected and control fibroblasts stimulated with SAG and quantified the ratio of GLI3 full length (GLI3FL) to repressor (GLI3R) forms by western blot analysis. We found that this ratio is increased two- to three-fold in DYNC2LI1 -mutant fibroblasts as compared with control cells ( Fig. 7d,e ). An increased ratio of GLI3FL to GLI3R suggests impaired proteolytic processing of GLI3, which has been proposed to be the underlying cause for the polydactyly commonly seen in SRPS and other ciliopathies [42] . In addition, total GLI3 was markedly increased in unstimulated DYNC2LI1 -mutant fibroblasts, implying that not only the processing is altered but also the total amount of available GLI3 is abnormal as well ( Fig. 7d,f ). To test whether this altered ratio had functional consequences on transcription of Hedgehog targets, we performed qRT–PCR of PTCH1 and GLI1 on control and SRPS fibroblasts. We found that both control and SRPS cells responded to SAG with an increase in PTCH1 and GLI1 cDNA ( Supplementary Fig. 5 ), suggesting that in these cells, the loss of the dynein-2 complex stability does not completely impair their ability to respond to SAG. Yet, altered GLI3FL to GLI3R ratios, together with the abnormal distribution of SMO into cilia of unstimulated SRPS cells, support impaired regulation of Hedgehog signalling in cells from SRPS cases with DYNC2LI1 mutations. We show that DYNC2LI1 mutations cause SRPS, expanding the number of genes associated with this condition. The phenotypic findings in these SRPS cases are similar to those seen in cases with DYNC2H1 (ref. 36 ) and WDR34 (ref. 13 ) mutations, supporting that these proteins are part of the same complex. Using SRPS fibroblasts, we show that DYNC2LI1 mutations result in loss of cilia length regulation, ciliary accumulation of IFT components and aberrant Hedgehog pathway activity. Rescue of mutant fibroblasts with human DYNC2LI1 corrected the cilia phenotype, directly confirming that the changes in cilia length and IFT resulted from the loss of normal DYNC2LI1. Our findings demonstrate that DYNC2LI1 is involved in both the repression of Hedgehog activity in the absence of stimulation and the activation of Hedgehog in response to stimulation. Alterations to Hedgehog signalling due to mutations in IFT-A proteins are typically mediated by either changes in cilia structure or trafficking, as opposed to non-ciliary functions of these proteins [43] . In the absence of stimulation, SMO is actively excluded from the cilia and GLI3 is processed into its repressor form. We show that SMO inappropriately enters the cilium in the absence of SAG stimulation in SRPS but not in control cells ( Fig. 7b ). This abnormal ciliary localization of SMO has been seen in other IFT mutants as well, including DYNC2H1 (ref. 41 ) and ICK [44] , and is suggestive of inappropriate Hedgehog pathway activation. Whether this SMO is active or not remains to be determined; however, the deficient processing of GLI3 into the repressor form suggests the former in DYNC2LI1 -mutant fibroblasts ( Fig. 7d,e ). We observed that DYNC2LI1 -mutant SRPS cells exhibit increased amounts of GLI3FL with and without stimulation, increased ratios of GLI3FL to GLI3R and decreased amounts of GLI3R upon stimulation as compared with controls. However, we could not identify a grossly abnormal transcriptional response in SRPS cells. This suggests that these cells can at least partially respond to Hedgehog signalling, though the in vivo consequences of persistent altered GLI3FL to GLI3R amounts in certain tissues, particularly in a temporal manner, may underlie developmental abnormalities, particularly polydactyly, as seen in these SRPS cases. We found that mutations in DYNC2LI1 do not preclude cilia formation, but rather cause cilia length dysregulation. On the basis of the phenotype of most mutants with diminished capacities for retrograde transport, including dynein-2 complex mutants, it is interesting that cilia in DYNC2LI1 mutants are longer than those in controls. In Chlamydomonas, dynein-2 null mutants (dhc1b [21] ; stf-1, stf-2 (ref. 22 )) have short, bulbous cilia with an accumulation of IFT-B components at their tips, suggesting an essential role for dynein-2 in recycling ciliary components back to the cell body. As IFT-B accumulates in these mutants, exhausting the pool of kinesin-2, the cilium loses its ability to grow or even maintain its length. In contrast, the DYNC2LI1 -mutant SRPS cases reported here have pronounced losses of both DYNC2H1 and DYNC2LI1 yet display robust ciliogenesis with longer-than-average cilia, despite having the characteristic IFT-B accumulations. This is similar to dynein-2 mutants in Tetrahymena (KO-D2LIC) [45] . It is thus likely that the DYNC2LI1 mutations alter the functioning of the dynein-2 complex without abolishing function altogether. The main defect in these cells appears to be loss of cilia length regulation as is evidenced by large variations in cilia lengths. It is possible that the small amount of remaining normal DYNC2H1 is enough to prevent the IFT congestion and stunted cilia seen in other mutants [46] . We therefore conclude that the residual activity of the dynein-2 complex in DYNC2LI1 -mutant fibroblasts was enough to support robust ciliogenesis but insufficient to ensure the correct regulation of primary cilium size. While we have shown that mutations in DYNC2LI1 produce a severe skeletal dysplasia, little is known regarding the expression of this gene in distinct tissues. qRT–PCR from RNA derived from a series of 16-week fetal tissues showed that DYNC2LI1 is expressed in all tissues studied, but is highest in bone ( Supplementary Fig. 3 ). Furthermore, the dynein-2 complex proteins we evaluated localized to the perichondrium/periosteum and primary spongiosa of bone ( Fig. 4 ), suggesting an important role in the developing skeleton. These regions have been shown to be important for signalling and organization of a normal cartilage growth plate [47] , [48] . The primary spongiosa, in particular, was reported to be irregular in SRPS cases with DYNC2H1 mutations [4] with loss of degradation of the mineralized hypertrophic zone, supporting the potential role of the dynein-2 complex in orchestrating the development of normal endochondral bone formation. Localization of the dynein-2 complex to the cartilage growth plate begins to provide insight into the reasons for altered endochondral ossification that are seen in SRPS. In summary, our findings establish the clinical and cellular consequences of DYNC2LI1 mutations and dynein-2 complex disruption in human primary cells, and support the profound importance of this protein complex in proper skeletogenesis. Exome sequencing Under an approved University of California at Los Angeles human subjects protocol, DNA was isolated and submitted to the University of Washington Center for Mendelian Genomics for library preparation and exome sequencing. The samples were barcoded, captured using the NimbleGen SeqCap EZ Exome Library v2.0 probe library targeting 36.5 Mb of genome, and sequenced on the Illumina GAIIx platform with 50 bp reads. Novoalign was used to align the sequencing data to the human reference genome (NCBI build 37) and the Genome Analysis Toolkit [49] was used for post processing and variant calling according to Genome Analysis Toolkit Best Practices recommendations [50] , [51] . Average coverage of targeted bases was × 103, × 61 and × 56 for R01-013A, R07-627A and R03-303A, respectively. For each sample, at least 90% of targeted bases were covered by at least 10 independent reads. Variants were filtered against dbSNP137, 95 NIEHS EGP exome samples (v.0.0.8), 6,503 exomes from the NHLBI Exome Sequencing Project (ESP6500), 1,000 genomes (release 3.20120430) and 40 in-house exome samples. Mutations were further compared with known disease-causing mutations in HGMD (2012.2). Variants were annotated using VAX [52] and mutation pathogenicity was predicted using the programs Polyphen [53] , Sift [54] , Condel [55] and CADD [56] . The mutations reported in this work were confirmed by bidirectional Sanger sequencing of amplified DNA from the proband and available parents ( Supplementary Fig. 1 ). Primer sequences used were: DYNC2LI1 -ex6 F: 5′-TTTTTGTTTTTGGGAGTCTTAGAA-3′; R: 5′-TTGCTGTAATTTTCCAGTGAACA-3′ DYNC2LI1 -ex12 F: 5′-ACCTGGCAGAATTGGAAGTG-3′; R: 5′-GGTGGGATGACAGGTGATTT-3′ DYNC2LI1 -ex13 F: 5′-GTGCTGCTTAGCCACACAGA-3′; R: 5′-GTGGGCACTTAACCTTGCAT-3′ Sequence trace files were aligned and analysed using Geneious version 7.1.4 created by Biomatters ( http://www.geneious.com/ ). The samples were part of a larger cohort of SRPS samples submitted for the purpose of identifying novel disease genes and characterizing the incidence of mutations in known genes. The cohort had not been previously tested for mutations in known SRPS-causing genes. Filtering strategy We assigned priority to mutations predicted to affect protein function (insertions or deletions, frameshifts, non-synonymous mutations and essential spice site mutations). We later included highly conserved splice region variants, allowing us to discover the DYNC2LI1 +3 splice site mutation. We assigned priority to mutations that had not been previously seen in the homozygous state in control databases and mutations with a minor allele frequency <0.005. Due to the recessive inheritance of SRPS, we looked for genes in which both alleles were potentially mutated. DYNC2LI1 stood out as a potential gene due to the incidence of unique, compound heterozygous mutations in three families in which the SRPS cases had strikingly similar X-ray features. RT–PCR RNA from SRPS case and control fibroblast cell lines was extracted using TRIZOL (Invitrogen 15596). RT–PCR was performed using SuperScript III One Step Kit (Invitrogen 12574-018) with the following DYNC2LI1 primers targeting a 431 bp template spanning exon 12: F: 5′-CGCTGTTTATCACAGCAGGA-3;′ R: 5′-CCAAGAAATCCAGCTTGTCC-3′. An amplified fragment of 431 bp corresponds to the wild-type RNA and a fragment of 339 bp corresponds to a transcript missing exon 12. Quantitative RT–PCR Total RNA was extracted from a series of 16-week fetal tissues as well as from control, R01-013A and R07-628A fibroblasts (with and without SAG treatment) using TRIZOL (Invitrogen 15596). cDNA was treated with DNAase (Invitrogen 18068) and reversed transcribed (Thermo Scientific K1621) according to the manufacturer’s instructions. qRT–PCR was performed with a real-time PCR detection system (Stratagene MX3005P) using SYBR Green PCR master mix (Thermo Scientific K0222) and standard thermocycler conditions. qRT–PCRs were performed in triplicate in a total volume of 25 μl for 3 independent replicates. Each sample was analysed for two housekeeping genes to normalize for RNA input amounts and to perform relative quantifications. Levels of transcripts in controls were set at 1. Melting curve analysis showed a single, sharp peak with the expected melting temperature for all samples. RT–PCR primers sequences were as follows: DYNC2LI1 F: 5′-GAAGGTGATGGAGCTGAAATTG-3′; R: 5′-GTATATTCCAAAGCTAAGGTTGGTT-3′ YWHAZ F: 5′-CAGCAGATGGCTCGAGAATA-3′; R: 5′-GAAGCATTGGGGATCAAGAA-3′ BACT F: 5′-TCCCTGGAGAAGAGCTACGA-3′; R: 5′-AGGAAGGAAGGCTGGAAGAG-3′ PTCH1 F: 5′-ACTCTGCTGGGAGTGCTGAT-3′; R: 5′-AAAACCAGCCCATTGAGAAC-3′ GLI1 F: 5′-ACACCGGTACCACTGTGTCC-3′; R: 5′-CGGCTGACAGTATAGGCAGA-3′ GAPDH F: 5′-CGTAGCTCAGGCCTCAAGAC-3′; R: 5′-GCTGCGGGCTCAATTTATAG-3′ GUSB F: 5′-CGAATCACTATCGCCATCAA-3′; R: 5′-CCCTTGGGATACTTGGAGGT-3′. Molecular cloning of DYNC2LI1 Human DYNC2LI1 cDNA (NM_016008.3) was synthesized using gBlock from IDT. The cDNA was flanked by XhoI and NotI restriction sites, which were used for insertion into pCAGIG, a pCAG-IRES-GFP vector (a gift from Connie Cepko (Addgene plasmid #11159)). The final construct was then used to express both untagged DYNC2LI1 and GFP in SRPS fibroblasts for the rescue experiments. Cell culture Unless otherwise stated, control and SRPS human fibroblasts from patients were grown in DMEM supplemented with 10% fetal bovine serum (FBS), 1% penicillin/streptomycin/ L -glutamine and were maintained at 37 °C with 5% CO 2 . For serum starvation and to promote ciliogenesis, cells were washed in PBS and incubated with serum-free media (or supplemented with 0.5% FBS) for 48 h. For stimulation of the sonic hedgehog pathway, serum-free media was supplemented with 500 nM SAG (Calbiochem 566660) for 24–48 h before cell fixation. hTERT–RPE1–GFP–CSAP cells (a kind gift from I. Cheeseman) [57] were grown in DMEM/F12 supplemented with 10% FBS, 1% penicillin/streptomycin and were maintained at 37 °C with 5% CO 2 . Rescue experiments Transfections of SRPS fibroblasts with h DYNC2LI1 IRES GFP were performed using Amaxa Kit for Primary Mammalian Fibroblasts according to manufacturer’s instructions and programme T-16. Twenty-four hours following transfection, cells were washed in PBS and incubated with serum-free media for an additional 48 h. RNAi For RNA-mediated interference, siGENOME (51626) Human DYNC2LI1 siRNA smartpool (Dharmacon) was employed against the following target sequences: 5′-GGAAUAAUAUGCCGAAGGA-3′ 5′-CAAAAGAUAUCGCUCACUU-3′ 5′-CCAUGUAGACAAAGUGAUA-3′ 5′-GGAAAGACUACUAUUAUUC-3′. Non-targeting siRNA was used as a control. RNAi was carried out using the Hiperfect reagent (Qiagen), according to the manufacturer’s instructions. Forty-eight hours following RNAi transfection, hTERT–RPE1–GFP–CSAP cells [57] (RPE1 cells with ciliary axoneme and centrioles marked by CSAP) were washed in PBS and incubated with an additional round of RNAi in serum-free media for 48 h to induce ciliogenesis. Knockdown was confirmed by western blotting. Immunofluorescence: cells were seeded into four-well chamber slides (LabTek) at a density of 4 × 10 4 cells per well and allowed to adhere overnight. After serum starvation, cells were washed twice with PBS and fixed in 95% methanol with 5 mM EGTA (pre-chilled to −20 °C) for 5 min. Alternatively, cells were fixed in 4% paraformaldehyde for 15 min at room temperature, washed and then permeabilized with 0.1% Triton-X-100 in PBS for 5 min at room temperature. After extensive washing, cells were blocked in PBS containing 5% serum for 1 h at room temperature. Primary antibodies were diluted in PBS containing 1–5% serum. Cells were incubated with the following primary antibodies for 1 h at room temperature or overnight at 4 °C: rabbit anti-WDR34 (1:200; Abcam ab81030), rabbit anti-DYNC2H1 (ref. 26 ; 1:150; Dynein HC2), rabbit anti-ARL13B (1:150; Proteintech 17711-1-AP), rabbit anti-IFT88 (1:150; Proteintech 13967-1-AP), rabbit anti-KIF3A (1:150; Sigma-Aldrich K3513), rabbit anti-TRAF3IP1 (1:100; Pierce PA5-30507), mouse anti-acetylated α-tubulin (1:2,000; 6-11B-1; Sigma-Aldrich T6793), rabbit anti-acetylated α-tubulin (1:800; D20G3; Cell Signaling Technology #5335), mouse anti-polyglutamylated tubulin (GluTUB; 1:300; Adipogen GT335), SMO (1:300; a kind gift from K. Anderson) and goat anti-GLI3 (10 μg ml −1 ; R&D Systems AF3690). After extensive washing, cells were incubated for 1 h at room temperature with Alexa Fluor 488/568-conjugated secondary antibodies (1:400; Invitrogen and Jackson ImmunoResearch) in PBS containing 5% serum. For rescue experiments in Figs 5d and 6b , Cy5- and Cy3-labelled secondary antibodies (1:400; Jackson ImmunoResearch) were used to detect ARL13B/IFT88 and GluTUB, respectively. Images were captured on an IX80 laser scanning confocal microscope (Olympus FV100 Spectral Confocal System) or a Leica Confocal TCS-SP2 using a × 100 1.40 numerical aperture or a × 63 (oil) objective 1.2 numerical aperture Images were collected with 1,024 × 1,024 pixel definition and Z-sections were taken at 0.5 μm step size. Max projections of the Z-stacks were used for primary cilium measurement and counting in ImageJ (NIH). To assess the impact of DYNC2LI1 mutations on ciliogenesis, we examined the localization of the ciliary membrane and axoneme markers ARL13B and glutamylated tubulin. ARL13B is a membrane protein belonging to the Arf family of GTPases that constitutively localizes to cilia. ARL13B signal is dispersed in the cytoplasm if a cell does not have a cilium, which allowed us to confidently score the percentage of ciliated cells when co-staining with an axonemal marker. Tubulin acetylation and glutamylation [58] are post-translational modifications associated with stable microtubule structures such as the cilia axoneme and, for glutamylated tubulin, the basal body and other centrioles. Quantification of IFT88 retention in the distal end of primary cilia was performed in similar-sized primary cilia using ImageJ (NIH). Polyglutamylated tubulin staining of centrioles and the proximal end of the axoneme served to determine the orientation of each primary cilium, allowing for the measurement of IFT88 signal intensity in the proximal end and in the remaining body of each primary cilium. After determining the ratio of IFT88 signal in each primary cilium, the resulting values were used to determine the average ratio of IFT88 signal for each experiment. Statistical analyses were performed with Prism v 5.0 (GraphPad). Immunohistochemistry A human humerus from a 14-week fetus was fixed in paraformaldehyde and decalcified with Immunocal for 2 days. After decalcification, samples were embedded in paraffin and 10 μm sections were prepared. Sections were treated with citrate buffer for antigen retrieval and quenched by peroxidase solution for 10 min each. Primary antibodies used were: rabbit anti-DYNC2LI1 (ref. 26 ; 1:200; LIC3), rabbit anti-WDR34 (1:150; Sigma HPA041091) and rabbit anti-DYNC2H1 (ref. 26 ; 1:150; Dynein HC2). After primary incubation, a Histostain Plus kit (Invitrogen 85-9243) was used for development with DAB. Protein/western blot analysis Cells were lysed in 1 × RIPA Buffer (Cell Signaling Technology) supplemented with 1 mM PMSF and a protease inhibitor cocktail (Sigma-Aldrich). Lysates were cleared by centrifugation (10 min at 16,000 g at 4 °C). A unit of 20–80 μg of protein per sample was loaded onto 10% or gradient SDS–polyacrylamide gels and separated by electrophoresis. Proteins were transferred to polyvinylidene difluoride or nitrocellulose membranes, which were then blocked with 5% milk for 1 h at room temperature. Membranes were then probed with primary antibodies diluted in 1–5% milk or BSA for 3 h at room temperature or overnight at 4 °C: rabbit anti-DYNC2LI1 (ref. 26 ; 1:200; LIC3), rabbit anti-WDR34 (1:200; Abcam ab81030), rabbit anti-DYNC2H1 (ref. 26 ; 1:150; Dynein HC2), rabbit anti-GAPDH (1:1,000; 14C10; Cell Signaling Technology #2118), mouse anti-γ-tubulin (1:10,000; GTU-88; Abcam ab11316), mouse anti-α-tubulin (1:5,000; Sigma T9026), and goat anti-GLI3 (1 μg ml −1 ; R&D Systems AF3690). After extensive washing, membranes were incubated with horseradish peroxidase-conjugated or fluorescent secondary antibodies and the signal was captured on film or in an Odyssey system (Licor). Protein amounts were quantified from scanned blots using ImageJ (NIH). Full scans of western blot data are included in Supplementary Fig. 6 . Accession codes: The sequence data have been deposited in ClinVar under the accession codes SCV000212251, SCV000212252, SCV000212253, SCV000212254, SCV000212255 and SCV000212256. How to cite this article: Taylor, S.P. et al . Mutations in DYNC2LI1 disrupt cilia function and cause short rib polydactyly syndrome. Nat. Commun . 6:7092 doi: 10.1038/ncomms8092 (2015).